Experimental evidence for the co-evolution of hominin tool-making teaching and language Hominin reliance on Oldowan stone tools—which appear from 2.5 mya and are believed to have been socially transmitted—has been hypothesized to have led to the evolution of teaching and language. Here we present an experiment investigating the efficacy of transmission of Oldowan tool-making skills along chains of adult human participants ( N =184) using five different transmission mechanisms. Across six measures, transmission improves with teaching, and particularly with language, but not with imitation or emulation. Our results support the hypothesis that hominin reliance on stone tool-making generated selection for teaching and language, and imply that (i) low-fidelity social transmission, such as imitation/emulation, may have contributed to the ~700,000 year stasis of the Oldowan technocomplex, and (ii) teaching or proto-language may have been pre-requisites for the appearance of Acheulean technology. This work supports a gradual evolution of language, with simple symbolic communication preceding behavioural modernity by hundreds of thousands of years. From 2.5 million years ago, early hominins were skilled stone knappers, capable of producing more than 70 sharp flakes from a single cobble core by striking it with a hammerstone (termed the Oldowan technocomplex [1] , [2] , [3] ; Fig. 1a , Supplementary Note 1 and Supplementary Figure 4 ). Existing remains show systematic flake detachment, maintenance of flaking angles and repair of damaged cores [4] . This complexity, along with present-day tool-making experiments [5] , implies that Oldowan technology was learned and required considerable practice [1] , [6] . Furthermore, the technology’s continual existence and wide geographic spread, along with hints of regional traditions [3] , [7] , indicate that it was socially transmitted, although the underlying psychological mechanisms remain poorly understood [8] . 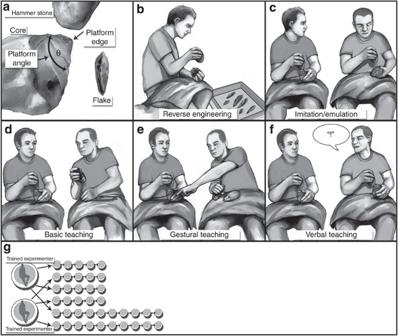Figure 1: Experimental design and structure. (a) A diagram of the stone knapping process. The hammerstone strikes the core with the goal of producing a flake. The platform edge and angle are important to the success of knapping. (b–f) The five learning conditions. (g) The structure of the experiment. For each condition, six chains were carried out (four short and two long); one of two trained experimenters started each chain (equally within each condition). Figure 1: Experimental design and structure. ( a ) A diagram of the stone knapping process. The hammerstone strikes the core with the goal of producing a flake. The platform edge and angle are important to the success of knapping. ( b – f ) The five learning conditions. ( g ) The structure of the experiment. For each condition, six chains were carried out (four short and two long); one of two trained experimenters started each chain (equally within each condition). Full size image Whether Oldowan stone tool making has implications for the evolution of human language and teaching (defined as active information donation [9] ) is debated [10] , [11] . Positions range from the view that Oldowan tool making indicates a major development in hominin cognition [8] , such as teaching or language [12] , to the hypothesis that chimpanzee-like emulation or imitation (reproducing the object manipulations or motor patterns of others, respectively) is sufficient to transmit knapping technology [13] . Accordingly, accounts of the evolution of language range from a gradual emergence beginning 2 mya (refs 14 , 15 ) to a relatively sudden appearance 50–100 kya (ref. 16 ). However, a difficulty with positing complex Oldowan communication is the apparent stasis in Oldowan technology for more than 700,000 years until Acheulean tools appear ~1.7 mya (refs 17 , 18 ). The absence of clear cultural change during this window seems inconsistent with the presence of language, and remains an outstanding mystery more generally [19] . Across disciplines, researchers are increasingly turning to gene-culture co-evolutionary accounts to explain the evolution of human cognitive abilities, including teaching and language [10] , [13] , [20] , [21] , [22] , [23] , [24] , [25] , [26] , [27] , [28] , [29] , [30] , [31] . Central to such hypotheses is the idea that cultural traits can both shape and be shaped by genetic evolution, and a number of examples of gene-culture co-evolution are now known from human evolution [26] , [27] , [28] , [29] , [30] . Hominin stone tool manufacture is a particularly interesting candidate case as the appearance of such technology 2.5 mya—at the dawn of Homo —and its continued deployment for millions of years, means it could have played a protracted role in human evolution. Furthermore, due to the challenging ecological niche that early hominins occupied [20] , [32] and the difficulty of acquiring tool-making skills [6] , fitness benefits were likely associated with the ability to make and deploy effective cutting tools [32] as well as the ability to rapidly transmit the skills [33] , and so a co-evolutionary relationship between tool making and cognition, specifically teaching and language, would seem plausible. Accordingly, Oldowan stone tool production could have generated selection for more complex forms of social transmission that enhanced the fidelity of information transmission. This could have resulted in a form of social transmission sufficient to transmit Acheulean technology reliably, and which would then generate selection for further increases in the complexity of social transmission, and so on. If this hypothesis is correct, changes in hominin cognition, including those underlying the appearance of Acheulean technology, could have depended upon selection generated by a reliance on Oldowan technology. In support of this hypothesis, archaeological remains show that changes to hominin morphology, including increased overall brain size, follow the advent of Oldowan tool making [3] . Other recent work has linked the cultural evolution of technologies to the capacity for high-fidelity social transmission [9] , [33] , [34] , [35] . However, hitherto such studies have either been theoretical or limited to somewhat artificial and abstract tasks. Accordingly, whether hominin lithic technology and social transmission genuinely represents a case of gene-culture co-evolution is currently unclear. Experiments with contemporary humans have provided insights into the cognitive and motor processes supporting lithic technology [23] , [24] , and could also establish which mechanisms support its transmission. However, research on the social transmission of tool making is very limited. For instance, a review of Acheulean tool making found that reduction strategies were highly consistent across individuals [36] . The authors suggest ‘true imitation’ (that is, reproducing the motor pattern of another individual through observational learning) is the minimal form of social transmission that could produce such consistency [36] . Furthermore, an unpublished experimental study found that ‘demonstrative gestures’ were sufficient for the co-operative procurement and initial reduction of bedrock slabs [37] . Only two studies have directly investigated the ability of contemporary adult humans to make tools following different means of social transmission, both comparing the efficacy of speech with symbolic gestural communication. One investigated the acquisition of Levallois technology [38] (a complex technology prevalent from 300–30 kya) and reported no differences between the conditions. However, the measure of performance was a binary (yes/no) assessment by the experimenter, leaving the possibility that more subtle differences existed but were undetected. The second investigated bifacial knapping [39] (a technique associated with Acheulean technology). Although the tools produced in both conditions showed similar shape, symmetry and quality, the two groups used different techniques, with verbally taught participants more accurately replicating the technique of the instructor (even though they lacked the skill to enact it effectively) [39] . As verbal and gestural communication are both symbolic forms of communication, further differences may yet emerge if a wider range of social transmission mechanisms, including imitation, emulation and subtle forms of pedagogy, are considered. This is particularly relevant to the manufacture of Oldowan technology, where the debate over the underlying transmission mechanisms is at its fiercest. Here we present a large-scale experimental study testing the capability of five social learning mechanisms to transmit Oldowan stone knapping techniques across multiple transmission events. By establishing the relative rates of transmission resulting from different means of communication, we aimed to provide insights into which forms of communication might have been selected for as a result of reliance on tool use. The mechanisms investigated are summarized as (i) reverse engineering, (ii) imitation/emulation, (iii) basic teaching, (iv) gestural teaching and (v) verbal teaching ( Fig. 1b–f ). In total, 184 participants took part, producing over 6,000 pieces of flint, each of which was weighed, measured and assessed for quality using a novel metric that we developed and verified. We find that, across six measures, performance increases with teaching and, particularly, language. However, there is little evidence that imitation/emulation enhances transmission. Our findings support a gene-culture co-evolutionary account of human evolution in which reliance on Oldowan tools would have generated selection favouring teaching and, ultimately, language. We suggest that Oldowan cultural evolution was limited, in part, by low-fidelity social transmission mechanisms. The appearance of Acheulean tools indicates the evolution of higher-fidelity social transmission, with teaching and/or some basic form of symbolic communication as plausible candidates. Accordingly, this work supports an early origin for language. Performance across conditions Across numerous measures of individual performance, we consistently found that teaching and language, but not imitation or emulation, enhanced the acquisition of stone knapping skills relative to reverse engineering (see Table 1 ). For instance, total flake quality only showed clear improvement with gestural or verbal teaching ( Fig. 2a ), with language nearly doubling performance relative to reverse engineering, and also improving performance relative to imitation/emulation and basic teaching. The number of viable flakes produced shows a similar pattern ( Fig. 2b ), with substantial increases relative to reverse engineering requiring gestural or verbal teaching. Moreover, unlike all forms of teaching, imitation/emulation did not increase the proportion of flakes that were viable ( Fig. 2c ). Neither was there evidence for an increase in the rate of manufacture of viable flakes with imitation/emulation; only verbal teaching was clearly associated with an increase ( Fig. 2d ). Similarly, only verbal teaching led to a clear increase (>30%) in the volume of core reduced ( Fig. 2e ). Finally, although there was no evidence that imitation/emulation increased the probability of a viable flake per hit, gestural teaching doubled and verbal teaching quadrupled this probability ( Fig. 2f ). Across the six measures there is strong evidence that verbal teaching increases performance relative to gestural teaching. Thus, teaching, but particularly verbal teaching, greatly facilitated the rapid transmission of flaking, whereas there is little evidence that imitation/emulation did so. Table 1 Effects of different transmission mechanisms on performance. 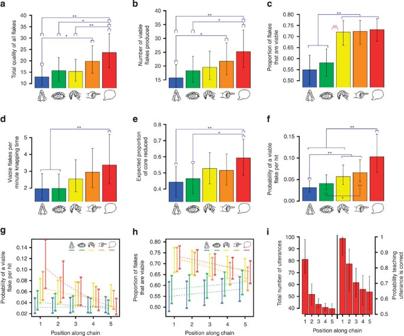Figure 2: Performance across conditions and along chains. Values shown are the median model estimates and the corresponding 95% central credible intervals. More complex forms of communication, in particular verbal teaching, increased several measures of participant performance, including (a) the total quality of all flakes, (b) the number of viable flakes, (c) the proportion of flakes that were viable, (d) the rate at which viable flakes were made, (e) the proportion of the core knapped and (f) the probability that each hit resulted in a viable flake. The brackets marked with double asterisks indicate contrasts for which there is strong evidence of a difference (95% credible interval excluding 0), single asterisks indicate cases for which there is weak evidence of a difference (90% credible interval excluding 0). The red bracket incindicates that the increase in performance from imitation/emulation to basic teaching is greater than the increase between all other adjacent conditions. (g,h) Although verbal and gestural teaching increased the probability of a viable flake per hit and the proportion of flakes that were viable, performance in these conditions decreased along chains such that across conditions performance was similar by position 5. With reverse engineering, performance did not decline along chains, suggesting it was already at floor levels. Position 1 corresponds to the first participant, not the trained experimenter. (i) With verbal teaching, both the total number of utterances (left hand bars) and the probability a teaching utterance was correct (right hand bars) decreased along chains. Key: reverse engineering: blue (n=37), imitation/emulation: green (n=34), basic teaching: yellow (n=38), gestural teaching: orange (n=37), verbal teaching: red (n=38). Full size table Figure 2: Performance across conditions and along chains. Values shown are the median model estimates and the corresponding 95% central credible intervals. More complex forms of communication, in particular verbal teaching, increased several measures of participant performance, including ( a ) the total quality of all flakes, ( b ) the number of viable flakes, ( c ) the proportion of flakes that were viable, ( d ) the rate at which viable flakes were made, ( e ) the proportion of the core knapped and ( f ) the probability that each hit resulted in a viable flake. The brackets marked with double asterisks indicate contrasts for which there is strong evidence of a difference (95% credible interval excluding 0), single asterisks indicate cases for which there is weak evidence of a difference (90% credible interval excluding 0). The red bracket in c indicates that the increase in performance from imitation/emulation to basic teaching is greater than the increase between all other adjacent conditions. ( g , h ) Although verbal and gestural teaching increased the probability of a viable flake per hit and the proportion of flakes that were viable, performance in these conditions decreased along chains such that across conditions performance was similar by position 5. With reverse engineering, performance did not decline along chains, suggesting it was already at floor levels. Position 1 corresponds to the first participant, not the trained experimenter. ( i ) With verbal teaching, both the total number of utterances (left hand bars) and the probability a teaching utterance was correct (right hand bars) decreased along chains. Key: reverse engineering: blue ( n =37), imitation/emulation: green ( n =34), basic teaching: yellow ( n =38), gestural teaching: orange ( n =37), verbal teaching: red ( n =38). Full size image Performance along chains In all conditions, as expected, performance decreased along chains relative to the trained experimenter as information was lost. However, with teaching, transmission was sufficiently improved that performance declined steadily along chains, whereas without teaching, the drop in performance along chains was so severe that performance immediately fell to floor levels (that is, the minimal level of performance we observed, likely representing participants’ intuitive understanding of stone knapping). For instance, with verbal teaching, the probability that each hit produced a viable flake ( Fig. 2g ), the number of viable flakes produced, and the proportion of flakes that were viable ( Fig. 2h ) all decreased steadily along chains, approaching the baseline performance observed with reverse engineering and imitation/emulation (see Table 2 ). Analyses of the utterances by participants in the verbal teaching condition showed that both the total number of utterances spoken and the proportion of teaching-related utterances that were correct also decreased along the chain ( Fig. 2i ). The rate of decline varied with topic, with knowledge of both the exterior platform angle and force-carrying ridges rapidly lost, but information concerning the platform edge being preserved for longer and with greater accuracy (see Table 2 ). Table 2 Effects of position along chains on performance. Full size table For a full listing of all model estimates, see Supplementary Tables 1–6 . The central finding of this work is that the social transmission of Oldowan technology is enhanced by teaching and, in particular, by language. This is in line with a gene-culture co-evolutionary account of human evolution and supports the hypothesis that Oldowan stone tool manufacture generated selection favouring increasingly complex teaching and language [13] , [24] , [40] . Although the learning period in this experiment (at 5 min long) is clearly unrealistically short compared with the length of time that Oldowan hominins likely had available to learn, particularly given available data showing that precise control of conchoidal fracture can take decades to acquire [41] and anthropological data showing that knapping skills are acquired across an apprenticeship lasting several years [42] , a short learning period is sufficient to examine the relative rates of transmission, which is the focus of this work. As such, we cannot rule out the possibility that with a longer learning period, performance across conditions would have converged. However, given that knapping skills are known to take years to develop fully [6] , [41] , we suspect that increasing the time spent learning would initially only increase the differences in performance across conditions, with any convergence only occurring after extensive learning. Given their magnitude, the observed differences in performance between conditions would likely translate into significant fitness differences in the shorter term. Key to our findings’ support of a gene-culture co-evolutionary account of human technology and cognition is the continuous improvement in the rate of transmission observed with increasingly complex forms of communication. For example, if verbal teaching provided transmission benefits, but simpler forms of teaching did not, then the co-evolutionary process would not be able to account for the evolution of these simpler forms of teaching. Likewise, if the transmission of tool making benefitted from simple teaching, but gained no further benefit from verbal teaching, then the co-evolutionary process would stop with simpler forms of teaching and could not explain the evolution of verbal teaching. Accordingly, our data imply that Oldowan tool making would have created a continuous selective gradient leading from observational learning to much more complex verbal teaching. This process need not have taken place entirely within the Oldowan, but was probably already underway during the Oldowan and likely continued well after, as Oldowan tools continued to be made for hundreds of thousands of years beyond the Oldowan time period. Furthermore, assuming that the transmission of more complex technologies also benefits from more complex means of communication, later technologies would have reinforced the gene-culture co-evolutionary dynamic. Such a process could have lasted for millions of years (and may be ongoing [29] ), with more complex communication allowing the stable and rapid transmission of increasingly complex technologies, which in turn generate selection for even more complex communication and cognition, and so forth. Although this places little necessary constraint on when teaching and language may have evolved, our central contribution is to provide evidence that Oldowan tools, produced by hominins since at least 2.5 mya, were involved in this dynamic. A second significant finding of this work is that the rate of transmission of Oldowan tool making is, at best, minimally enhanced by the addition of imitation/emulation relative to reverse engineering. That the low level of performance with imitation/emulation and reverse engineering is stable along chains (and that performance with teaching and language collapses to this level) suggests a baseline level of performance reliant on little transmitted knowledge, and which could well be achieved through intuition and individual trial-and-error learning. We suggest that the rapid decline of performance with teaching and language to this baseline merely reflects the short learning time employed in this study. Previous transmission chain studies have established that periods of individual practice can bolster the stability of socially transmitted knowledge [43] . This suggests that with more time to learn, with bouts of teaching and language integrated with periods of individual practice, the benefits of teaching and language would likely have been preserved for longer. Likewise, a benefit of observational learning relative to reverse engineering may well appear over a longer learning period. However, our data suggest that any such benefit is likely to be less than the benefit that would be derived through teaching across a similar timespan because of the improved rate of transmission with teaching. Accordingly, although we do not suggest that imitation is insufficient to transmit the technology per se , our findings support other recent work in implying that observation alone is an inefficient means to acquire stone tool-making skills [23] , [44] , [45] . Limited information concerning tool manufacture can, no doubt, be rapidly acquired through imitation or emulation; for instance, the basics of core, hammerstone or flake selection [36] , the requirement to strike the core with the hammerstone and some idea of the force are required. However, it seems plausible that the rapid striking action associated with tool manufacture hinders the transmission of more subtle information crucial to knapping, such as details of the point of percussion or the platform edge and angle, through observation alone. It is here that teaching (for example, slowing down the striking action, pointing to appropriate targets, demonstrating core rotation, manual shaping of pupil’s grasp) and verbal instruction likely provide immediate benefits to the pupil. Indeed, transcripts from the verbal teaching condition show that abstract knapping concepts, such as the platform angle, were transmitted between individuals in the verbal teaching condition (see Supplementary Fig. 3 ). It may well be the capacity for arbitrary labels such as ‘platform angle’ that facilitates transmission with verbal teaching; such labels break the task into constituent parts, can be used to identify the important elements and provide a clear framework with which pupils can go on to teach others. Language not only allows transmission of the skill itself, but also the ability to transmit the skill to others effectively. Third, our findings have implications for one of the most enduring puzzles of human evolution: the apparent stasis of the Oldowan technocomplex, which lasted 700,000 years [8] , [11] , [19] , [45] . Our experiment suggests that Oldowan technological change could have been restricted by low-fidelity forms of social transmission that prevented the spread of innovations. This suggestion is supported by the slow spread of Oldowan technology across Africa, which indicates that this technology was difficult for Oldowan hominins to transmit [3] . Furthermore, the acquisition of Oldowan knapping skills is not trivial even for modern humans, as shown by our finding that the benefits of teaching and language were rapidly lost in transmission. Although we cannot conclusively identify what form Oldowan transmission might have taken, our data indicate imitation or emulation as likely candidates. In naturalistic contexts, the relatively poor transmission that we observed with imitation and emulation could well be too slow and imprecise for innovations to be transmitted reliably, leaving the technology unable to increase in complexity until more effective communication had evolved. The suggestion that low-fidelity social transmission is a limiting factor on technological development might contribute to an understanding of why human culture is so complex compared with the behavioural traditions of non-human animals [46] , [47] . Although human social transmission has allowed the cumulative elaboration of a vast number of technologies and behaviours, non-human animal social transmission has not. It seems possible that this is because non-human animal social transmission, which appears to be largely limited to forms of observational learning less sophisticated than those of humans [43] , lacks the fidelity required to transmit more complex innovations, thus constraining cumulative cultural evolution [34] , [35] , [48] . Even the modest knapping ability of extensively trained bonobos [49] , [50] may rely on their prior training in symbolic communication [51] . Although it is plausible that a similar co-evolutionary process has operated to a lesser degree in some other species, such as other apes [52] , it remains an open question as to why their tool use did not generate selection for the higher-fidelity social transmission (teaching and language) observed in humans. One possibility is that the technologies of other apes are either sufficiently simple that they can be acquired through more basic mechanisms or so hard to acquire that they can only rarely be transmitted successfully, removing the benefit to teaching [9] . Task difficulty might also explain a previous experimental finding that simple transmission mechanisms were sufficient for cumulative cultural evolution in the context of human paper-plane design [53] ; this task may be sufficiently simple that teaching is of little benefit. Alternatively, ape reliance on tool use could be insufficient for the benefits of tool-use to outweigh the costs of complex social transmission, thus preventing teaching from increasing fitness [9] . Any of these constraints would undermine selection for higher-fidelity social transmission, hindering the co-evolutionary process. Given that our findings support a co-evolution of Oldowan tool use and complex communication, it might seem puzzling that the Oldowan stasis should last so long. If the selective advantage was present, why did more complex communication not evolve for 700,000 years? A likely explanation is that more complex communication may well have evolved during the Oldowan, but that this alone was insufficient for the evolution of stone tool technology. The appearance of Acheulean tools may have additionally been contingent on the evolution of other aspects of cognition, such as technical comprehension or the hierarchical planning of actions [54] , [55] , [56] , as well as demographic and socio-ecological factors [57] , [58] . Accordingly, the extraordinary length of the Oldowan stasis could indicate that a large number of limiting factors needed to be overcome before innovations could appear and spread. Given this, our findings imply that the appearance of Acheulean tools 1.7 mya (refs 17 , 18 ) reflects, in part, the evolution of mechanisms of transmission that facilitated the more effective transmission of Oldowan tool-making, but also enabled the reliable transmission of the sub-goals and techniques required to make the distinctive and regularly shaped Acheulean tools [59] . We cannot specify the form of this transmission with precision. However, given the observation that chimpanzees are capable of some form of observational learning, yet cannot produce stone tools approaching the quality of the earliest known Oldowan examples [13] , combined with the complexity of Acheulean technology [36] , we suggest that teaching in the form of facilitated observation (similar to our basic teaching condition) is the minimal plausible form of social transmission for Acheulean hominins and that rudimentary forms of language are a possibility. However, although our findings suggest that Oldowan hominins would have benefitted from modern language, the suggestion that modern language evolved during the Oldowan seems unlikely given how slowly technology evolved thereafter. This leaves open the possibility that the transmission of Acheulean technology was reliant on a form of (gestural or verbal) proto-language [12] , [60] , [61] . This need not imply that Acheulean hominins were capable of manipulating a large number of symbols or generating complex grammars. Our findings imply that simple forms of positive or negative reinforcement, or directing the attention of a learner to specific points (as was common in the gestural teaching condition), are considerably more successful in transmitting stone knapping than observation alone. This is supported by existing theoretical work that suggests positive and negative feedback greatly enhances the rate of transmission [33] . Whether or not simple symbolic communication was present during the Acheulean, we anticipate that the gene-culture co-evolutionary dynamic between tools and communication was, and that it would continue beyond the Acheulean, generating selection favouring the use of symbols for increasingly subtle and abstract concepts, and contributing to the eventual evolution of modern language capabilities. In sum, our data support the hypothesis that a gene-culture co-evolutionary dynamic between tool use and social transmission was on-going in human evolution, starting at least 2.5 mya and potentially continuing to the present. The simplicity and stasis of Oldowan technology are indicative of a limited form of social transmission, such as observational learning, that only allowed the transmission of the broadest concepts of stone knapping technology. Whatever its nature, this was sufficient to support limited transmission among individuals with prolonged contact, but insufficient to propagate innovations more rapidly than they were lost, and would have contributed to the stasis in the Oldowan technocomplex. However, hominin reliance on stone technology would have generated selection for increasingly complex communication that allowed the more effective spread of stone-tools. Under this continued selection, teaching, symbolic communication and eventually verbal language may have been favoured, allowing the ready transmission of abstract flaking concepts, such as the role of the exterior platform angle in choosing where to strike [38] , which our findings shown are effectively transmitted by language. Given the increased complexity of the later Acheulean and Mousterian lithic technologies, with their reliance on ‘long sequences of hierarchically organized actions’ [36] , [38] and other abstract concepts, our results imply that hominins possessed a capacity for teaching—and potentially simple proto-language—as early as 1.7 mya. Participants and materials One hundred and eighty-four participants took part in the study. This sample size was chosen based on effect sizes observed in previous transmission chain studies. Participants were students at the University of St Andrews recruited through the University’s experimental sign-up system. Across the experiment, we used 2 tonnes of Brandon flint from Norfolk, UK, broken up into cores of roughly 1 kg. We also used 100 granite hammerstones collected from the coastline near Stonehaven, Scotland. Experimental design Adult human participants ( N =184) first learned, were tested on their ability, and then helped others to learn, to knap stone flakes using a granite hammerstone and flint core, across five cumulatively complex transmission conditions (see Fig. 1b–f ): (i) Reverse Engineering: pupils were provided with a core and hammerstone for practice, but saw only the flakes manufactured by their tutor and not their tutor themselves; (ii) Imitation/Emulation: in addition to having their own core and hammerstone, pupils also observed their tutor making flakes, but could not interact with them; (iii) Basic Teaching: in addition to demonstrating tool production, tutors could also manually shape the pupil’s grasp of their hammerstone or core, slow their own actions and reorient themselves to allow the pupil a clear view (this condition replicates teaching reported in non-human primates [62] ); (iv) Gestural Teaching: tutors and pupils could also interact using any gestures, but no vocalizations and (v) Verbal Teaching: tutors and pupils were also permitted to speak. Participants were assigned to conditions at random and blinding was not possible. The test given to participants to assess their ability was to make as many good-quality flakes as possible from a single core. This reflected pressures on hominin knappers to make the most of the limited availability of high-quality knapping materials. Participants were arranged into transmission chains [63] in which information was passed along chains of participants, with each participant learning from the previous participant and acting as tutor to the next participant. For each condition, we carried out four short chains (≤5 participants) and two long chains (≤10 participants) per condition (see Fig. 1g ). Experimenters trained in stone knapping (T.J.H.M. and N.T.U.) acted as tutor to the first participant. To ensure participant motivation, we paid participants between £10 and £20, with the value dependent upon their performance when tested. In the teaching conditions (conditions 3–5), participants’ payment was also dependent upon how well their pupils went on to perform; thus tutors were motivated to teach effectively. In the imitation/emulation condition (condition 2), participants’ payment was also dependent upon how well they performed when demonstrating, this was to motivate demonstrators to focus on their own performance and not to teach the pupil. Procedure Upon arrival, participants were briefed on the experimental procedure and their consent was required to proceed (ethical approval was given by St Andrews UTREC, code: BL6376). Before they learnt to knap, and to ensure that participants understood what Oldowan tools were used for, participants were given an information sheet, flint flakes of varying quality, chamois leather and wooden sticks. They were then given 5 min to use these items to gain an understanding of what made a good-quality sharp cutting flake. The information sheet gave only very brief information on the history and uses of Oldowan stone tools, and not any information as to how to make them beyond striking a flint core with a hammerstone. The learning/teaching period lasted for 5 min, after which participants were interrupted. After the learning phase, the pupil then advanced to the test phase. Participants were instructed to take as long as they needed for the test phase, however, if they had not stopped within 18 min, the experimenter encouraged them to finish and after 20 min the experimenter instructed them to stop (only 12.5% of participants used the full 20 min). After the test phase (if applicable), participants went on to teach the next pupil. Once the procedure was complete, participants were debriefed and paid before leaving. Data All flints used by participants were bagged throughout the experiment. In total, participants produced 6,214 pieces of flint greater than 2 cm in diameter. All of these pieces were weighed, measured and assessed for viability (that is, whether they had possible use as a cutting tool) and quality (using a novel metric, which we developed, that took into account flake mass, cutting edge length and diameter; see Supplementary Methods for details). Any pieces less than 2 cm across were not coded, as 2 cm was considered to be the minimum size for a flake to possibly have utility as a butchery tool [64] . We also weighed participants’ cores both before and after knapping. Participants’ behaviour during the experiment was recorded using video cameras and we subsequently measured the length of time participants spent knapping and the number of times participants struck their core with their hammerstone. We also transcribed everything participants said while in the verbal teaching condition and split it into utterances ( N =1,481) for analysis. In particular, all utterances were coded as either ‘correct’ or ‘incorrect’, which was determined relative to established knapping practices. The robustness of flake viability ratings, as well as video coding, was tested by triple and double coding, respectively, a subset of the data. In both cases, the level of agreement between coders was very high (see Supplementary Methods for details of the double/triple coding procedure). Analyses We analysed the data using Bayesian GLMMs fitted using MCMC methods in OpenBUGS [65] , [66] . We modelled six different measures of individual performance: (i) the number of viable flakes produced, (ii) the total quality of flakes produced, (iii) the proportion of flakes that were viable, (iv) the rate at which viable flakes were produced, (v) the probability of a viable flake per hit and (vi) the proportion of their core successfully reduced. These measures were modelled as a function of condition, position along the chain, interactions between condition and position, initial core mass and random repeat-level effects. For a full description of the experimental procedure and all analyses, see Supplementary Methods . For a comparison of the model results with the raw data, see Supplementary Figs 1 and 2 . How to cite this article : Morgan, T. J. H. et al. Experimental evidence for the co-evolution of hominin tool-making teaching and language. Nat. Commun. 6:6029 doi: 10.1038/ncomms7029 (2015).